Tuning the acoustic frequency of a gold nanodisk through its adhesion layer To fabricate robust metallic nanostructures with top-down patterning methods such as electron-beam lithography, an initial nanometer-scale layer of a second metal is deposited to promote adhesion of the metal of interest. However, how this nanoscale layer affects the mechanical properties of the nanostructure and how adhesion layer thickness controls the binding strength to the substrate are still open questions. Here we use ultrafast laser pulses to impulsively launch acoustic phonons in single gold nanodisks with variable titanium layer thicknesses, and observe an increase in phonon frequencies as a thicker adhesion layer facilitates stronger binding to the glass substrate. In addition to an all-optical interrogation of nanoscale mechanical properties, our results show that the adhesion layer can be used to controllably modify the acoustic phonon modes of a gold nanodisk. This direct coupling between optically excited plasmon modes and phonon modes can be exploited for a variety of emerging optomechanical applications. Coherent coupling schemes between photons and phonons make it possible to effectively bridge the fields of photonics and phononics, both of which are important for information signalling and storage. For example, ultrasensitive optomechanical devices employing Fabry–Perot type optical cavities with an oscillating end mirror as the mechanical resonator have recently been realized to detect the quantum limit of coherent coupling between single photons and single phonons [1] , [2] , [3] , [4] , [5] , [6] , [7] . Transfer of optical momentum into mechanical motion occurs through the pressure exerted by the photons on the oscillating cavity mirror: the photon pressure-induced mechanical motion of the mirror changes the cavity length and is detected optically. Dynamic back action, controlled by a feedback loop, can produce damping or amplification of acoustic motion depending on laser frequency [1] , [2] , [8] , [9] . Optomechanically induced transparency windows have also been achieved [10] , [11] . For strong coherent optomechanical coupling, high finesse optical cavities and high-quality factor mechanical oscillators are typically needed to obtain the requisite long photon survival times and to overcome the thermal and mechanical losses of the oscillator. For plasmonic nanostructures, optomechanical coupling and excitation of coherent phonon modes can be realized directly through optical excitation because of the large resonant absorption cross-sections associated with the surface plasmon resonance, a collective oscillation of the conduction band electrons. Strong absorption coupled with the impulsive heating that follows optical excitation by ultrafast laser pulses makes it possible to launch coherent acoustic vibrations in the nanostructure. Using time-resolved transient extinction spectroscopy, these acoustic phonon modes can be probed optically, as the mechanical deformations of the nanostructure shift the plasmon resonance. This method enables one to obtain a direct picture of the mechanical properties of the nanostructure that would otherwise be impossible to detect by more traditional methods [12] , [13] , [14] , [15] , [16] , [17] , [18] , [19] , [20] , [21] , [22] , [23] , [24] , [25] , [26] , [27] , [28] , [29] , [30] , [31] , [32] , [33] , [34] , [35] , [36] , [37] . With this approach, the surface plasmon of the metal nanostructure leads first to a hot electron distribution, which then couples to the lattice within a time period much shorter than the motion of its constituent atoms, launching coherent lattice vibrations—acoustic phonons—in the nanoparticle [38] . Because of the greatly different timescales of electron motion (femtoseconds) compared with atomic displacements (picoseconds), optomechanical coupling in plasmonic nanostructures is typically an incoherent process. However, a very recent study has shown that coherent control is possible through clever nanostructure design and a 2-pump excitation scheme [39] , making it potentially possible to design active feedback mechanisms between plasmonic and mechanical oscillators constructed from a single nanostructure. Significant research efforts have been focused on the study of acoustic phonon modes in metallic nanoparticles using both ensemble [12] , [13] , [14] , [15] , [16] , [17] , [18] , [19] , [20] , [21] , [22] , [23] , [24] , [25] , [26] and single-particle [23] , [27] , [28] , [29] , [30] , [31] , [32] , [33] , [34] , [35] , [36] transient extinction measurements. These studies have shown that the elastic constants of the nanoparticles, obtained from the measured lattice vibrations, agree well with those of the corresponding bulk materials, suggesting that, generally speaking, there is no change in the elastic properties of nanoscale objects because of their smaller size [40] . However, vibrational properties strongly depend on absolute size, shape and surrounding environment of nanoparticles [40] . Precise control over the dimensions of nanostructures fabricated using top-down lithography [41] is typically required for device applications that take advantage of coherent phonon modes. For lithographically fabricated nanostructures, an adhesion layer such as Cr or Ti is almost universally used to strongly bind Au to substrates such as glass or Si, for example, because of the inert chemical nature of Au [42] , [43] . While both Cr and Ti are used, Ti is often more favourable than Cr for optical applications because it provides a larger transmittance [44] . Currently, the factors that control adhesion between substrate and nanostructure are not well understood: the common practice of depositing 2- to 3-nm-thick Ti adhesion layers in the case of Au is entirely empirical. Only a single study, where Cr/Au nanorings lithographically fabricated on a glass substrate were investigated using ultrafast transient extinction spectroscopy, showed that the observed breathing mode frequencies likely depend on the Cr adhesion layer. They observed that the experimental vibrational frequencies of the Cr/Au nanorings were intermediate to those predicted by models assuming entirely free and entirely fixed structures [30] . These results suggest that the adhesion layer facilitates some degree of substrate binding, and also indicates that ultrafast transient extinction spectroscopy may be a useful method for further investigating this property. With a more detailed understanding of how this interfacial layer affects mechanical properties, it may be possible to controllably tune the acoustic modes, in addition to the adhesion strength, of the nanostructure. This capability would be highly desirable for enabling altogether new applications that exploit this optically addressable link between the plasmonic and the mechanical properties of nanostructures. In this work, we show that the Ti adhesion layer thickness not only controls the mechanical coupling of a gold nanodisk to a substrate, but by varying its nanometre-scale thickness, it can be tuned between the two extreme cases of a free nanostructure and a nanostructure rigidly attached to the underlying substrate. These results are obtained on lithographically prepared individual Au nanodisks of varying height, diameter and Ti adhesion layer thickness, probing the breathing mode frequency optically by means of ultrafast transient extinction spectroscopy. We also observe a linear increase in the lattice vibration frequency with Ti volume ratio, suggesting that the coherent lattice vibration could be used as an accurate and sensitive tool for probing the metal composition by entirely noninvasive means. 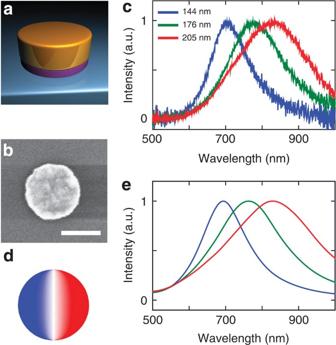Figure 1: Characterization of single Au nanodisks. (a) Schematic cross-section of an Au nanodisk. Blue, magenta and gold represent the glass substrate, Ti adhesion layer and Au nanodisk, respectively. (b) SEM image of a Au nanodisk with a diameter of 176 nm. Scale bar, 100 nm. (c) Scattering spectra of Au nanodisks with diameters of 144 nm (blue), 176 nm (green) and 205 nm (red) with sizes referring to the diameter of the bottom of the nanodisk. The thickness of the Au and Ti layers were 35 and 1.5 nm, respectively. (d) Simulated charge plot of the fundamental in-plane plasmon mode of the Au/Ti nanodisk. (e) Simulated scattering spectra of Au/Ti nanodisks having the same dimensions as inc. Fabrication and characterization of single Au nanodisks Au/Ti nanodisks were fabricated using electron-beam (e-beam) lithography (see Methods, Supplementary Table 1 ). Figure 1a shows an illustration of a 35-nm-thick nanodisk with a Ti adhesion layer of 1.5 nm deposited on a glass coverslip. Ti and Au thicknesses were controlled by the deposition rate and time as monitored by a quartz crystal microbalance in the deposition chamber. The final thickness of the nanodisk was verified by atomic force microscopy (AFM) and agreed well with the value reported by the microbalance ( Supplementary Fig. 1 ). Scanning electron microscopy (SEM) imaging of an individual Au/Ti nanodisk with a diameter of 176 nm in an array of 20 nanodisks separated by 10 μm revealed a diameter variation of less than 2% ( Fig. 1b ). A side-view SEM image of the nanodisk shows that the top of the nanodisk was ∼ 10% smaller than the bottom of the nanodisk ( Supplementary Fig. 2a ). From these measurements, we estimate an idealized tilt angle of the nanodisk sidewall to be 75° ( Supplementary Fig. 2b ). Figure 1: Characterization of single Au nanodisks. ( a ) Schematic cross-section of an Au nanodisk. Blue, magenta and gold represent the glass substrate, Ti adhesion layer and Au nanodisk, respectively. ( b ) SEM image of a Au nanodisk with a diameter of 176 nm. Scale bar, 100 nm. ( c ) Scattering spectra of Au nanodisks with diameters of 144 nm (blue), 176 nm (green) and 205 nm (red) with sizes referring to the diameter of the bottom of the nanodisk. The thickness of the Au and Ti layers were 35 and 1.5 nm, respectively. ( d ) Simulated charge plot of the fundamental in-plane plasmon mode of the Au/Ti nanodisk. ( e ) Simulated scattering spectra of Au/Ti nanodisks having the same dimensions as in c . Full size image To correctly assign the fundamental mode of the lattice vibration, nanodisks with diameters of 144, 176 and 205 nm were fabricated and measured using conventional dark field microscopy (see Methods, Fig. 1c ). The plasmon resonance red shifts with increasing diameter due to an increase in aspect ratio (diameter/height), similar to nanorods, illustrating that the surface plasmon oscillation is parallel to the substrate. Finite difference time domain (FDTD) simulations were performed using the actual dimensions and compositions of the nanodisks on a semi-infinite glass substrate including the actual light excitation and collection geometries (see Methods). These simulations confirm that the in-plane plasmon mode originates from the bi-layered Au/Ti structure. The simulated spectra ( Fig. 1e ) agree well with the experimental results, indicating that Ti and Au do not form an alloy. The charge distribution of a nanodisk calculated at the plasmon resonance peak with in-plane polarized incident light displays a dipole pattern ( Fig. 1d ), validating the assignment of an in-plane plasmon mode. This determination is critical for the correct identification and interpretation of the observed acoustic vibration mode. Acoustic vibration mode of single Au nanodisks Single-particle transient extinction spectroscopy was utilized to investigate the acoustic vibrations of the nanodisks ( Supplementary Fig. 3 ). Femtosecond pump and probe pulses were generated with a 86-MHz repetition rate, unamplified Ti:sapphire oscillator with the fundamental laser wavelength set to λ =820 nm. Frequency-doubling yielded pump pulses at λ =410 nm where interband transitions in the Au nanodisks are excited to create hot electrons that after coupling to the lattice are responsible for launching coherent acoustic vibrations. Pulses at λ =820 nm were used as a probe to detect small changes in transmittance near the surface plasmon resonance maximum. The nanodisks were specifically designed to support surface plasmon resonances at this probe wavelength. The pump and probe beams were collinearly overlapped and tightly focused on the sample through an oil-immersion objective mounted on a custom-built microscope. Transients of the pump induced extinction changes for a single nanodisk were then acquired by positioning a single nanodisk within the area of the probe beam and changing the time delay between pump and probe beams (see Methods). Scattering spectra were taken before and after the transient extinction measurements ( Supplementary Fig. 4 ) and showed no change because of potential laser-induced damage of the nanodisks, when low pump (66 μW, 0.76 pJ per pulse) and probe (22 μW, 0.25 pJ per pulse) powers were used. Indeed, using a two-temperature model (see Supplementary Note 3 ) [45] , the induced lattice temperature due to the pump and probe beams was only 396 K. The time transient of a single nanodisk shows a damped harmonic oscillation because of the excitation of coherent acoustic vibrations ( Fig. 2a ). These acoustic vibrations can be probed optically because changes in the Au dielectric function due to electron occupancy and nanoparticle expansion lead to shifts and broadening in the plasmon resonance [46] . 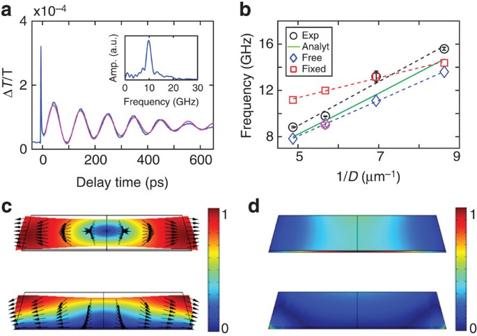Figure 2: The acoustic vibration mode of single Au nanodisks. (a) Time transient of a single 176-nm diameter Au nanodisk (blue) with Au and Ti thicknesses of 35 and 1.5 nm, respectively. Fit with equation (1) is also shown (magenta). Inset: Fourier Transform analysis of experimental transient. (b) Acoustic vibration frequencies of single nanodisks as a function of 1/D, whereDis the nanodisk diameter. Au and Ti thicknesses were held constant. The error bars of the experimental data points (black circles) represent the s.d. for each nanodisk size determined from measurements of at least five nanostructures. The magenta data point corresponds to Au nanodisks without a Ti adhesion layer. Experiments are compared with simulations based on an analytical model (green line) and FEM simulations based on a free surface model (blue diamonds) and fixed surface model (red squares). See text for details. The lines are fits to the simulated data. The slopes and intercepts are summarized inSupplementary Table 2. (c) FEM simulations of the displacement fields using a free surface model (top) and a fixed surface model (bottom). A cross-sectional view of the nanodisk is presented, where arrows indicate the direction of the displacement field and thin black lines represent the unperturbed shape of the nanodisk. The colour scale bar represents the normalized displacement field. (d) Corresponding volumetric strain fields for the free and fixed cases inc. The colour scale bar represents the normalized volume strain field. The frequency of the acoustic vibration can be extracted either by Fourier transform analysis, or by fitting the data following the fast initial decay directly using the following equation [34] , [35] : Figure 2: The acoustic vibration mode of single Au nanodisks. ( a ) Time transient of a single 176-nm diameter Au nanodisk (blue) with Au and Ti thicknesses of 35 and 1.5 nm, respectively. Fit with equation (1) is also shown (magenta). Inset: Fourier Transform analysis of experimental transient. ( b ) Acoustic vibration frequencies of single nanodisks as a function of 1/ D , where D is the nanodisk diameter. Au and Ti thicknesses were held constant. The error bars of the experimental data points (black circles) represent the s.d. for each nanodisk size determined from measurements of at least five nanostructures. The magenta data point corresponds to Au nanodisks without a Ti adhesion layer. Experiments are compared with simulations based on an analytical model (green line) and FEM simulations based on a free surface model (blue diamonds) and fixed surface model (red squares). See text for details. The lines are fits to the simulated data. The slopes and intercepts are summarized in Supplementary Table 2 . ( c ) FEM simulations of the displacement fields using a free surface model (top) and a fixed surface model (bottom). A cross-sectional view of the nanodisk is presented, where arrows indicate the direction of the displacement field and thin black lines represent the unperturbed shape of the nanodisk. The colour scale bar represents the normalized displacement field. ( d ) Corresponding volumetric strain fields for the free and fixed cases in c . The colour scale bar represents the normalized volume strain field. Full size image where τ a is the decay time for thermal coupling to the environment, τ b is the damping time of the lattice vibrations, ν is the vibration frequency, A and B are amplitudes and φ is a phase factor. The absolute amplitudes of the acoustic vibrations are more complicated to determine because changes in the real and imaginary parts of the Au dielectric function need to be extracted from plasmon resonance shifts and broadening [46] , [47] , requiring more than the one probe wavelength that is used here and is typical for single-particle studies with low pulse energy, high repetition rate lasers to avoid photo-induced damaging of the nanostructures. The magenta curve in Fig. 2a is a fit to the experimental data using equation (1), yielding ν =9.8 GHz with a damping time of τ b =410 ps. Fourier transform analysis applied to the same data also gives ν =9.8 GHz ( Fig. 2a , inset). Measurements of the acoustic vibrations of other nanodisks within the same array over different days gave a s.d. of ∼ 3% for the extracted acoustic vibration frequency. This value is consistent with the nanodisk size variation of 2%. This high degree of reproducibility, limited by the resolution of the e-beam fabrication process, allowed us to resolve differences in acoustic vibration frequencies on the order of 0.5 GHz. A linear relationship between the acoustic vibration frequency and the inverse diameter of the nanodisk confirms that we are exciting the two-dimensional, in-plane breathing mode ( Fig. 2 ). For a nanodisk, both the extension and breathing modes, where the phonons vibrate along axial and radial directions, respectively, can be excited. According to the linear elastic theory, the vibrational frequencies of extensional and breathing modes are inversely proportional to the height and the diameter of the nanodisk, respectively ( Supplementary Equation (1) in Supplementary Note 1 ) [16] , [48] , [49] . To identify the breathing mode, nanodisks with diameters of 116, 144, 176 and 205 nm were fabricated on the same glass substrate to ensure that the thickness was identical for all structures, that is, 1.5 and 35 nm for Ti and Au, respectively. Single-particle transient extinction measurements were performed on these nanodisks, and the acoustic vibration frequencies were obtained by fitting the data to equation (1). Indeed, a linear relationship between the acoustic vibration frequency and the reciprocal diameter is obtained ( Fig. 2b ), allowing us to assign the observed acoustic vibrations to an in-plane breathing mode, while the extension mode is not observed. These experimental results are compared with an analytical model (green line in Fig. 2b ) based on linear elastic theory for free bimetallic nanodisks with dimensions and composition derived from the experimental values ( Supplementary Note 2 ). Compared with the experimental results, the analytical model correctly predicts the slope, but consistently underestimates the values of the breathing mode frequency for all nanodisks. The analytical model neglects the influence of the glass substrate, but includes the change in the stiffness of the nanodisk as it explicitly includes the Ti layer. This disagreement between experiment and theory must then be caused by an interaction of the nanodisks with the underlying substrate, as the breathing mode frequency of an Au nanodisk with a diameter of 176 nm without the Ti layer agrees quantitatively with the analytical model (magenta symbol in Fig. 2b ). The presence of the Ti adhesion layer causes a blueshift of the breathing mode because of mechanical coupling with the substrate ( Fig. 2 ). To investigate this Ti layer-mediated coupling further, the acoustic vibration of a Au/Ti composite nanodisk on a glass substrate was simulated for two extreme cases: (1) the free surface case, where the bottom surface of the Ti remains free from the substrate; and (2) the fixed surface case, where the bottom surface of Ti is rigidly fixed to the glass substrate. An analysis of these two cases was performed using the finite element method (FEM, see Methods). The normalized displacement fields of a Au/Ti nanodisk for the free surface case (top) and for the fixed surface case (bottom) are shown in Fig. 2c , whereas the corresponding volumetric strain fields are given in Fig. 2d . For the free surface case, the radial displacement of the nanodisk is homogeneous from bottom to top of the nanodisk, as there is no adhesion between the Ti layer and the glass substrate. In contrast, for the fixed surface case, the Ti layer is rigidly clamped to the substrate and less displacement is observed for the bottom portion of the nanodisk than for its free surface. Interestingly, we observe that the greatest volumetric strain for the free surface case occurs in the thin Ti layer at the nanodisk base; the volumetric strain exhibits a discontinuity at the interface between the two metals because of their difference in Poisson’s ratio. This result is simply because of the lower Poisson’s ratio of Ti relative to Au that ensures greater variation in volume; for the limiting case of an incompressible solid (Poisson’s ratio of 1/2), no change in volume would occur. The corresponding breathing mode frequencies as a function of the inverse diameter were also obtained using the FEM simulations for the free surface and the fixed surface cases ( Fig. 2b ). An increase in breathing mode frequency with decreasing nanodisk diameter is seen for both models, with the values from the fixed surface case all being larger than for the free surface case. However, the experimental slope agrees better with the slope from the free surface model, which is in excellent agreement with the analytical model. The fact that our experimental data agree more closely with the free surface case suggests that for a 1.5-nm adhesion layer, the nanodisks are only weakly bound to the glass substrate. Effect of Ti layer thickness on nanodisk acoustic frequency The results in Fig. 2 strongly suggest that the acoustic vibration frequency of a Au/Ti nanodisk is a function of Ti adhesion layer thickness. To investigate this possibility, Au nanodisks of 35 nm height were fabricated on top of Ti layers with thicknesses varying between 0 and 4 nm. The measured and simulated scattering spectra again agree well ( Supplementary Fig. 5 ), confirming a bilayer configuration. The breathing mode frequencies of a single Au/Ti nanodisk without a Ti adhesion layer, and with a 2-nm Ti adhesion layer, are 9.2 and 10.6 GHz, respectively ( Fig. 3a ). The results for all Au/Ti nanodisks are summarized in Fig. 3b . Here we see that the acoustic vibration frequency increases linearly with Ti thickness, suggesting that increasing Ti layer thickness corresponds to an increasingly stronger adhesion to the glass substrate. On the basis of a pump power dependence ( Supplementary Fig. 6 ), we can rule out temperature-induced changes in the Au elastic constants as a possible alternative explanation [50] . We can also eliminate the possibility that changes in the total height of the nanodisk with increasing Ti layer thickness could be responsible for the observed frequency shift ( Supplementary Note 4 ). Measurements on pure Au nanodisks with thicknesses of 25, 35 and 45 nm ( Supplementary Fig. 7 ) as well as 15, 25 and 35 nm nanodisks with a 2-nm Ti layer ( Supplementary Fig. 8 ) all showed red shifts of the phonon frequencies, opposite to the trend shown in Fig. 3b . 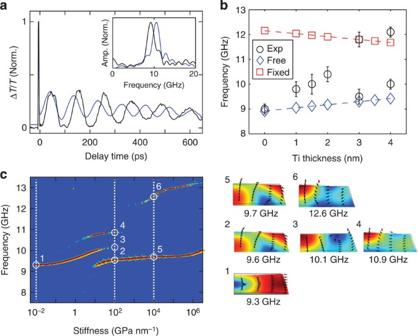Figure 3: Effect of Ti adhesion layer thickness on the nanodisk acoustic vibration frequency. (a) Time transients of single nanodisks with Ti thickness of 2 (blue) and 0 (black) nm and the same Au thickness of 35 nm. Insets: Fourier transform analysis with colours corresponding the time transients in the main panel yielding frequencies of 9.2 and 10.5 GHz, respectively, in agreement with the values obtained from equation (1), that is, 9.2 and 10.6 GHz. (b) Breathing mode frequencies as a function of Ti thickness where the Au thickness is constant at 35 nm. The error bars of the experimental data points (black circles) represent the s.d. for each different nanodisk determined from measurements of at least five nanostructures. The experimental data points are compared with FEM simulations assuming a free surface model (blue diamonds) and fixed surface model (red squares), where the lines are linear fits to the simulated data. The slopes and intercepts are summarized inSupplementary Table 3. (c) FEM simulations illustrating the dependence of acoustic modes on the stiffness of a coupling layer introduced to model the binding strength between the nanodisk and the substrate. The diameter of the nanodisk is 176 nm and the Ti and Au thicknesses are 3 and 35 nm, respectively. Left: Contour plot highlights the frequencies with the maximal volume changes in the bimetallic nanodisk. Right: displacement fields (1–6, referenced in the contour plot) with the maximal volume changes for a few representative modes at three different values of the coupling layer stiffness. Figure 3: Effect of Ti adhesion layer thickness on the nanodisk acoustic vibration frequency. ( a ) Time transients of single nanodisks with Ti thickness of 2 (blue) and 0 (black) nm and the same Au thickness of 35 nm. Insets: Fourier transform analysis with colours corresponding the time transients in the main panel yielding frequencies of 9.2 and 10.5 GHz, respectively, in agreement with the values obtained from equation (1), that is, 9.2 and 10.6 GHz. ( b ) Breathing mode frequencies as a function of Ti thickness where the Au thickness is constant at 35 nm. The error bars of the experimental data points (black circles) represent the s.d. for each different nanodisk determined from measurements of at least five nanostructures. The experimental data points are compared with FEM simulations assuming a free surface model (blue diamonds) and fixed surface model (red squares), where the lines are linear fits to the simulated data. The slopes and intercepts are summarized in Supplementary Table 3 . ( c ) FEM simulations illustrating the dependence of acoustic modes on the stiffness of a coupling layer introduced to model the binding strength between the nanodisk and the substrate. The diameter of the nanodisk is 176 nm and the Ti and Au thicknesses are 3 and 35 nm, respectively. Left: Contour plot highlights the frequencies with the maximal volume changes in the bimetallic nanodisk. Right: displacement fields (1–6, referenced in the contour plot) with the maximal volume changes for a few representative modes at three different values of the coupling layer stiffness. Full size image The lattice frequency shift caused by the increase in Ti thickness clearly originates from a stronger binding between the nanodisk and the substrate. To further substantiate this conclusion, FEM simulations of nanodisks with different Ti thicknesses were performed using the free and fixed surface models. In these simulations, the Ti thickness was varied from 0 to 4 nm, while the diameter and Au thickness of the nanodisks were 176 and 35 nm, respectively, for all nanostructures. The blue and red symbols in Fig. 3b indicate the results of these simulations. The acoustic vibration frequencies of the nanodisks using the free surface model are always lower than those obtained with the fixed surface model, independent of Ti thickness. In the case without a Ti layer, the measured acoustic vibration frequency matches well with the simulated frequency of the free surface model, consistent with the fact that, in the absence of a Ti layer, Au is known to adhere poorly to glass substrates. With increasing Ti thickness, the measured frequencies increase, deviating from the free surface model and approaching values of the fixed surface model for a Ti thickness of 3 nm. Further increase to a Ti thickness of 4 nm has little effect, supporting the empirical observations that maximal adhesion of a Au nanostructure to a substrate could be achieved using at least a 3-nm Ti layer. This result demonstrates an increase in binding strength between Au and the glass substrate when the Ti thickness is increased through the range of 0–4 nm, from the nonbinding to the strong binding regimes for e-beam-fabricated metal nanostructures. Interestingly, for the nanodisks with a 3- or 4-nm Ti layer, the breathing mode splits into two frequencies as shown in Fig. 3b (see also Supplementary Fig. 9 ). This splitting of the acoustic vibration mode is due to the strong mechanical coupling between the nanostructure and the substrate [39] . To theoretically investigate the origin of the observed frequency splitting, we introduce a thin coupling layer of varying stiffness between the bimetallic nanodisk and the glass substrate in the FEM simulations (see Methods). As identification of the dominant mode excitement is required here, FEM simulations and analysis were performed in a similar manner to the pump-probe measurements. Namely, a step change in the temperature was applied to the bimetallic nanodisk/substrate system, and the resulting volumetric change in the nanodisk was calculated. This volumetric change is directly related to the change in nanodisk electron density, which dictates the change in plasmon resonance [16] . Bulk material and thermal properties of Au, Ti and glass were used. The frequency response of this change in volume, as a function of the substrate stiffness, is presented in Fig. 3c (left) as a contour plot—only contours describing the maximal changes in volume are shown, which dominate the experimental response. This analysis yields identical frequencies and modes to those in Fig. 2 for the completely free and rigidly fixed cases (dominant mode identification in these limits is trivial). The results in Fig. 3c (left) can therefore be directly compared with the measurements. As the stiffness increases, several different acoustic modes emerge as shown in Fig. 3c (right), which also illustrates the corresponding displacement fields at three different stiffness values (marked 1–6 in Fig. 3c ). For a small stiffness (10 −2 –1 GPa nm −1 ), that is, weak coupling, we observe only one dominant mode and its acoustic frequency increases with increasing stiffness of the coupling layer, consistent with the experimental results for Ti layer thicknesses in the range of 0–2 nm. Furthermore, the simulated displacement field at an acoustic frequency of 9.3 GHz corresponding to 10 −2 GPa nm −1 is same as the one simulated with the free surface model ( Fig. 2c ). As the stiffness is increased, multiple other acoustic modes start to appear. At 10 4 GPa nm −1 the two dominant acoustic modes have frequencies of 9.7 and 12.6 GHz, closely matching the values measured for the nanodisk with a 3-nm Ti layer. These FEM results clearly demonstrate that the frequency splitting arises from a stronger coupling between the bimetallic nanodisk and the glass substrate. The frequencies of the acoustic breathing mode increase with Ti thickness, as the mechanical coupling between the Au and the glass substrate is strengthened. In particular, we observed a full range of adhesion coupling, from nonbinding to complete adhesion for a minimum Ti layer thickness of 3 nm. Furthermore, we found that a Ti adhesion layer of a given thickness enables stronger binding to the surface than a Cr adhesion layer. Au nanodisks with a diameter of 176 nm and a height of 35 nm were fabricated using Cr adhesion layers with thicknesses of 3 and 6 nm and investigated by transient extinction spectroscopy ( Supplementary Fig. 10 ). Only one acoustic vibration frequency at 10.6 GHz is observed for the nanodisks with a 3-nm Cr layer. This frequency is lower than the value expected from the fixed surface model. When the Cr adhesion layer thickness is increased to 6 nm, two acoustic frequencies are again measured with the value of the higher frequency mode matching the fixed surface model, similar to the behaviour discussed in Fig. 3 for Au nanodisks with 3- and 4-nm Ti adhesion layers. These results suggest that, unlike Ti, a 3-nm Cr layer is not thick enough for complete adhesion of the Au nanodisks to the glass substrate. Single-particle measurements of the acoustic vibrations are essential for determining the homogeneous damping time and its variation among different Au/Ti nanodisks within the same sample in order to gain insight into the dissipation of the mechanical oscillations as a function of Ti adhesion layer thickness. Ensemble measurements strongly underestimate the intrinsic damping time as even slightly different nanostructure dimensions within a inhomogeneous collection of nanoparticles yield a corresponding distribution of acoustic frequencies, which when summed up lead to an apparent faster damping of the harmonic oscillation [13] , [23] . The total damping time of an acoustic vibration originates from (1) the mechanical coupling between the nanodisk and the substrate, (2) the acoustic impedance mismatch between the nanodisk and the environment and (3) intrinsic damping mechanisms such as lattice defects [31] , [34] . Contributions from impedance mismatch can be ruled out because transient extinction measurements were performed in air [31] , [34] . In addition, because all nanodisks were fabricated using the same method, we expect that, despite the inherent polycrystalline nature of nanodisks produced by e-beam lithography, lattice defects within the Au layer are similar for all samples. The experimental dependence of the homogeneous damping time and its distribution suggests that the nature of the Au–glass and Au–Ti interfaces plays a dominant role in the decay of the acoustic vibrations. 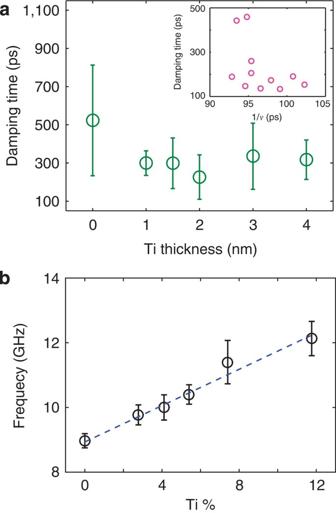Figure 4: Homogeneous damping time and acoustic frequency of bimetallic Au/Ti nanodisks. (a) Damping time of the acoustic vibration as a function of Ti adhesion layer thickness. Inset: damping time versus inverse frequency for individual nanodisks with Au and Ti thicknesses of 35 and 2 nm, respectively. Note that for the samples with 3- and 4-nm Ti adhesion layers the damping times for the low- and high-frequency modes are almost identical and only the latter are shown here. (b) Acoustic vibration frequency of single Au/Ti nanodisks as a function of Ti volume percentage. Data for the nanodisks with 3- and 4-nm Ti adhesion layers are not included here because of the splitting of the acoustic vibration frequency into two modes caused by the strong binding to the substrate. The dotted blue line is a linear fit to the data points. The error bars of the experimental data points ina,brepresent the s.d. for each different nanodisk determined from measurements of at least five different nanostructures. Figure 4a plots the homogeneous damping time as a function of Ti adhesion layer thickness. Apart from an increase in damping time without a Ti layer, consistent with weaker mechanical coupling to the glass substrate, a similar dependence on Ti thickness as found for the acoustic vibrations ( Fig. 3b ) is not obvious considering the large error bars—these represent the s.d. from measurements performed on different nanodisks on the same sample. Considering that (i) the error from repeated measurements of the same nanodisk is much smaller than the one shown in Fig. 4a (9% versus 52% for the nanodisks with 2 nm Ti and 35 nm Au layers) and (ii) no correlation exists between the damping time and the inverse acoustic frequency ( Fig. 4a inset) and hence the nanodisk size (spread <2%), we conclude that the large variations in the damping times are likely due to differences in the Au–glass and Au–Ti interfaces. This conclusion is consistent with previous studies on samples prepared by e-beam lithography [13] , [30] . A similar behaviour is also observed for the quality factor Q = πντ b ( Supplementary Fig. 11 ) and the relative oscillation amplitudes ( Supplementary Fig. 12 ). Figure 4: Homogeneous damping time and acoustic frequency of bimetallic Au/Ti nanodisks. ( a ) Damping time of the acoustic vibration as a function of Ti adhesion layer thickness. Inset: damping time versus inverse frequency for individual nanodisks with Au and Ti thicknesses of 35 and 2 nm, respectively. Note that for the samples with 3- and 4-nm Ti adhesion layers the damping times for the low- and high-frequency modes are almost identical and only the latter are shown here. ( b ) Acoustic vibration frequency of single Au/Ti nanodisks as a function of Ti volume percentage. Data for the nanodisks with 3- and 4-nm Ti adhesion layers are not included here because of the splitting of the acoustic vibration frequency into two modes caused by the strong binding to the substrate. The dotted blue line is a linear fit to the data points. The error bars of the experimental data points in a , b represent the s.d. for each different nanodisk determined from measurements of at least five different nanostructures. Full size image Interestingly, the results of the Au–Ti nanodisks studied here can be combined in a single graph by plotting the breathing mode frequencies as a function of Ti volume percentage ( Fig. 4b ). We find a linear relationship between the Ti% and the breathing mode frequencies of the 176-nm-diameter Au–Ti nanodisks, independent of the thicknesses of the individual Au and Ti layers where the total height varied from 17 to 37 nm. Theoretically, in the limit of high aspect ratio nanodisks (height<<diameter), the acoustic breathing frequencies are expected to depend solely on the ratio of Ti-to-Au thicknesses (that is, Ti%), consistent with the measurements in Fig. 4b for our moderately thin particles. According to Fig. 4b , the acoustic frequency of supported Au nanodisks can be tuned over a 3-GHz range through their Ti adhesion layer. This general relationship also suggests that it is possible to determine the Ti% and therefore the Ti thickness for a known total height of an e-beam fabricated nanostructure with nanometre resolution using the noninvasive optical method of ultrafast transient extinction spectroscopy. The Ti% also affects the maximum and linewidth of the plasmon resonance [51] , [52] , [53] . However, quantitative extraction of the Ti% from extinction spectra is more complicated if the nanostructure dimensions are altered as well because of spectral changes arising from geometry-governed intrinsic plasmonic properties such as the nanodisk aspect ratio in our case. No such limitation applies in Fig. 4b where the acoustic vibration frequencies scale linearly with Ti % independent of Ti and Au thickness. This conclusion is further supported by the plasmon resonance maxima and linewidths extracted from FDTD-simulated extinction spectra for nanodisks with the same dimensions and compositions as in Fig. 4b ( Supplementary Fig. 13 ). In conclusion, the lattice vibrations of lithographically fabricated Au nanodisks were investigated as a function of Ti adhesion layer thickness using single-particle transient extinction spectroscopy. Our results point towards a straightforward method for tuning the acoustic phonon frequency of a nanostructure in the GHz range by controlling the thickness of its adhesion layer, a new variability that may lead to new types of plasmon-based optomechanical applications. The GHz frequency is important for wireless communication, remote sensing and radar in civilian, military and government applications for such diverse areas as weather monitoring, air traffic control, logistics tracking, payment and anticounterfeit measures [54] , [55] . In addition, our study provides direct insight into the adhesion layer thickness-dependent mechanical coupling between a transparent support substrate and plasmonic nanostructures fabricated by e-beam lithography. Single-particle measurements of the homogeneous damping time, furthermore, reveal the heterogeneous nature of the metal–substrate interface. The insight provided here with respect to the mechanical properties of substrate-supported nanoscale materials is central to nonlinear photoacoustic imaging [56] , [57] , micro- and nanomechanical resonators [58] , [59] and microbalances [60] , [61] , [62] , [63] , [64] . Sample preparation Individual gold nanodisks were fabricated on a glass substrate using e-beam lithography. The substrates were sonicated in acetone for 5 min, cleaned with oxygen plasma for 5 min and spin-coated with a layer of polymethyl methacrylate resist (PMMA 950 A2, MicroChem) and Espacer 300Z (Showa Denko). E-beam patterning of the resist was performed using a FEI QUANTA 650 SEM with a voltage of 30 K and a beam current of 40 pA. Ti adhesion and Au layers were deposited on the substrates by e-beam evaporation. The thickness of the deposited films was monitored by a quartz crystal microbalance and further confirmed by AFM measurements. The structures were treated with a standard lift-off process via incubation in N-methyl-2-pyrrolidone at 65 °C for 2 h. Dark field scattering spectroscopy Scattering spectra of individual nanodisks were measured by a dark field microscope. The white light source was focused on the sample by a × 50 dark field objective with a numerical aperture (N.A.) of 0.55, and the scattered signals were collected by the same objective and directed into a spectrograph (Princeton Instruments Acton 2156i) towards a CCD (charge-coupled device) camera (Pixis 400 BR). The spectrum was obtained by dividing the collected signal by the white light spectrum after subtracting the background noise. Single-particle transient extinction spectroscopy A diode-pumped laser (Coherent) was used to pump a Ti-Sapphire laser (KMLab, Griffin) to generate a 820-nm beam with a pulse duration of ∼ 80 fs. The 410-nm pump beam was generated by frequency-doubling of part of the 820-nm fundamental beam in a Barium boron oxide crystal (Altos). The 410-nm pump and 820-nm probe beams were split by a dichroic mirror and the probe beam passed through an optical delay line. The intensity of the pump beam was modulated by an acousto-optic modulator (IntraAction) with a frequency of 400 kHz. The pump and probe beams were recombined by another dichroic mirror before being focused on the sample by an objective (Zeiss, N.A.=1.4). The pump and probe powers were 66 and 22 μW, respectively, unless mentioned specifically. The diameter of the probe beam was 400 nm. The pump and probe beams were collected by a second objective (Zeiss, N.A.=0.6) and passed through a 750-nm long-pass filter so that only the probe beam was detected by a photodiode (Femto). The signal was fed into a lock-in amplifier and connected to a counterboard (National Instruments). Transient extinction images, used to locate individual nanodisks, were obtained with pump and probe beams overlapped temporarally by scanning the sample through the focused laser beams using a piezo scanning stage (Phyisk Intrumente). Time transients were acquired by moving the optical delay line and repeated at least two times to ensure the reproducibility of each measurement. FEM modelling Supplementary Equation (3) in Supplementary Note 2 was implemented in the commercial finite element modelling software COMSOL Multiphysics, using its eigenfrequency solver. We have considered two limiting cases. In the first case the bottom surface of the titanium disk was kept free and in the second case the bottom surface of the titanium disk was rigidly fixed, that is, no displacement. We therefore covered the limiting cases where the substrate does not affect disk motion, and where the substrate rigidly restrains the disk. For numerical simulations, symmetry in the nanodisks allowed the computational domain to be reduced to the r – z plane only, where the z -direction was along the thickness of the disk, r was along the radius of the disk and the origin was in the centre of the bottom surface of the titanium layer. This geometry is illustrated in Supplementary Fig. 14 for a bimetallic disk. The reported results are independent of mesh size to within 0.1%. To demonstrate the influence of the substrate, we have used the frequency response solver of COMSOL Multiphysics. A thin layer of varying stiffness was considered to produce different coupling strengths between the bimetallic nanodisk and the glass substrate. To truncate the thickness of the thicker glass layer, a perfectly matched layer (PML) on the bottom of the glass substrate was used to absorb propagating acoustic waves. The dimensions of the glass layer and the PML were optimized by considering different thicknesses and radii of these layers. Finite different time domain simulation Simulations were performed using the finite-difference time-domain method-based software Lumerical FDTD Solution. This method solved the time-dependent Maxwell’s equation. An individual Au nanodisk with a Ti adhesion layer on a semi-infinite SiO 2 substrate was surrounded by PMLs. The dielectric constants were adopted from ref. 65 for Au and from ref. 66 for Ti and SiO 2 . The geometric parameters for the Au nanodisks were adopted from the SEM images. The mesh size on the disk was 0.5 nm. For the remaining environment, the maximum mesh size was 26 nm. To calculate the scattering and absorption spectra, we recorded the net power flow scattered from the disks and into the disks. How to cite this article: Chang, W.-S. et al. Tuning the acoustic frequency of a gold nanodisk through its adhesion layer. Nat. Commun. 6:7022 doi: 10.1038/ncomms8022 (2015).